Regulation of NF-κB signalling by the mono-ADP-ribosyltransferase ARTD10 Adenosine diphosphate-ribosylation is a post-translational modification mediated by intracellular and membrane-associated extracellular enzymes and many bacterial toxins. The intracellular enzymes modify their substrates either by poly-ADP-ribosylation, exemplified by ARTD1/PARP1, or by mono-ADP-ribosylation. The latter has been discovered only recently, and little is known about its physiological relevance. The founding member of mono-ADP-ribosyltransferases is ARTD10/PARP10. It possesses two ubiquitin-interaction motifs, a unique feature among ARTD/PARP enzymes. Here, we find that the ARTD10 ubiquitin-interaction motifs bind to K63-linked poly-ubiquitin, a modification that is essential for NF-κB signalling. We therefore studied the role of ARTD10 in this pathway. ARTD10 inhibits the activation of NF-κB and downstream target genes in response to interleukin-1β and tumour necrosis factor-α, dependent on catalytic activity and poly-ubiquitin binding of ARTD10. Mechanistically ARTD10 interferes with poly-ubiquitination of NEMO, which interacts with and is a substrate of ARTD10. Our findings identify a novel regulator of NF-κB signalling and provide evidence for cross-talk between K63-linked poly-ubiquitination and mono-ADP-ribosylation. ARTD10 (formerly PARP10) [1] , originally identified as a MYC-interacting protein, possesses mono-adenosine diphosphate (ADP)-ribosyltransferase activity [2] , [3] . The ARTD family consists of 18 members. Although they share a conserved catalytic domain, they can be divided into three classes depending on their catalytic activity [1] . Members of the first class can generate and modify their substrates with polymers of ADP-ribose (PAR). The best-studied class 1 enzyme is ARTD1 (formerly PARP1). The second class contains mono-ADP-ribosyltransferases, with ARTD10 being the founding member, while members of the third class possess no catalytic activity [1] , [3] , [4] . PARylation regulates various cellular processes, such as DNA repair, specific signalling processes and gene transcription [5] . The functional consequences of PARylation are mediated by distinct protein domains, including macrodomains, WWE (named after two conserved tryptophan residues and a glutamate residue) and PAR-binding zinc-finger (PBZ) domains [6] , [7] , [8] , [9] , [10] . In contrast to the function of class 1 ARTD enzyme-mediated PARylation, little is known about the biological relevance of mono-ADP-ribosyltransferases. ARTD10 is capable of mono-ADP-ribosylating itself and core histones [2] , [3] , but its biological relevance remains undefined. Within the ARTD family, ARTD10 is the only member with two ubiquitin-interaction motifs (UIMs). UIMs are one kind of a number of distinct ubiquitin-interaction domains [11] , [12] . These exert multiple functions, in part dependent on their binding to different poly-ubiquitin (pUb) species [13] . For example, K48-pUb marks proteins for proteasomal degradation. In contrast K63-pUb functions as a scaffold in signalling processes, including the nuclear factor-κB (NF-κB) signal transduction pathway [14] , [15] , [16] . NF-κB controls many key processes, such as proliferation and cell survival, and is important in regulating inflammation and tumorigenesis among others [17] , [18] . We have found that the UIMs of ARTD10 interact with K63-pUb chains. We have addressed whether and how ARTD10 communicates with NF-κB signalling. In response to the chemokines interleukin-1β (IL-1β) or tumour necrosis factor-α (TNFα), tumour-necrosis factor receptor-associated factor (TRAF) proteins are activated some of which function as K63-specific E3 ubiquitin ligases [17] . Several downstream effectors are modified with or bind to K63-pUb, promoting activation of the TAB/TAK kinase complex and, further downstream, the IκB kinase (IKK) complex [19] . As a consequence NF-κB transcription factors translocate into the nucleus and regulate target gene expression. Thus, distinct pUb chains are key post-translational modifications in controlling the flow of information in the NF-κB signalling pathway [20] . The findings that we report here suggest that ARTD10 regulates NF-κB signalling by interacting with K63-pUb. This interferes with the activation of NF-κB, inhibits the translocation of p65 into the cell nucleus and results in reduced target gene expression. Mechanistically ARTD10 prevents the K63-pUb of NEMO, which is a substrate of ARTD10. Together these findings suggest that mono-ADP-ribosylation (mADPr) is a novel post-translational modification that impinges on NF-κB signalling and cross-talks with K63-pUb. ARTD10 UIMs bind specifically to pUb chains Several protein domains with possible functional relevance have been identified in ARTD10 (ref. 2 ). Unique among the ARTD family members are two UIMs in the C terminal half of ARTD10 ( Fig. 1a ) [2] , [11] , [12] . They are functional because GST-ARTD10(600–868), containing both UIMs, bound K63-pUb that was at least tetrameric ( Fig. 1c ). No other tested ubiquitin species were bound. The interaction was specific because GST-ARTD10(600–868)-ΔUIM, in which key amino acids involved in ubiquitin binding were substituted ( Fig. 1b ), did not bind ( Fig. 1c ). Mutating UIMs individually resulted in reduced binding ( Fig. 1d ), suggesting that both UIMs contributed to the interaction with K63-pUb. It is worth noting that mutating the UIMs did not affect ARTD10 catalytic activity ( Fig. 1e ). Thus, the UIMs of ARTD10 have the capacity to interact with specific ubiquitin polymers. 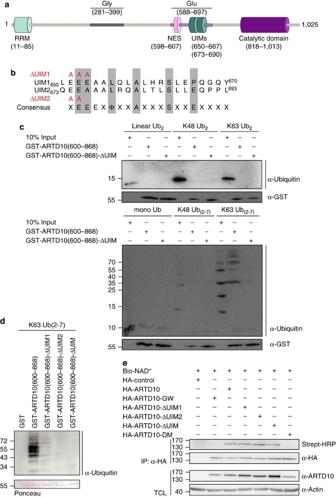Figure 1: The ubiquitin-interaction-motifs (UIMs) of ARTD10 bind specifically to ubiquitin polymers. (a) Schematic diagram of ARTD10 with its functional domains. (b) The sequences of both UIMs are shown in comparison with a UIM consensus sequence. Substitutions of conserved amino acids in UIM1 and UIM2 are indicated. (c) GST-ARTD10(600–868) and GST-ARTD10(600–868)-ΔUIM with both UIMs mutated (b) were incubated with the indicated ubiquitin proteins. Ubiquitin bound to the GST fusion proteins was analysed by immunoblotting. (d) The interaction of K63-linked poly-ubiquitin with the indicated GST-ARTD10 fusion proteins was determined in pull-down assays followed by immunoblotting. (e) Haemagglutinin (HA)-tagged ARTD10 or mutants were expressed transiently in HeLa cells, lysed in TAP-lysis buffer and the proteins were immunoprecipitated using HA-specific antibodies. ADP-ribosylation assays were performed using biotinylated NAD+(50 μM). Protein levels were visualized using HA-specific antibodies, the automodification of ARTD10 was determined by streptavidin-HRP on western blots. Glu, glutamate-rich region; Gly, glycine-rich region; NES, nuclear export sequence; RRM, RNA-recognition motif. Figure 1: The ubiquitin-interaction-motifs (UIMs) of ARTD10 bind specifically to ubiquitin polymers. ( a ) Schematic diagram of ARTD10 with its functional domains. ( b ) The sequences of both UIMs are shown in comparison with a UIM consensus sequence. Substitutions of conserved amino acids in UIM1 and UIM2 are indicated. ( c ) GST-ARTD10(600–868) and GST-ARTD10(600–868)-ΔUIM with both UIMs mutated ( b ) were incubated with the indicated ubiquitin proteins. Ubiquitin bound to the GST fusion proteins was analysed by immunoblotting. ( d ) The interaction of K63-linked poly-ubiquitin with the indicated GST-ARTD10 fusion proteins was determined in pull-down assays followed by immunoblotting. ( e ) Haemagglutinin (HA)-tagged ARTD10 or mutants were expressed transiently in HeLa cells, lysed in TAP-lysis buffer and the proteins were immunoprecipitated using HA-specific antibodies. ADP-ribosylation assays were performed using biotinylated NAD + (50 μM). Protein levels were visualized using HA-specific antibodies, the automodification of ARTD10 was determined by streptavidin-HRP on western blots. Glu, glutamate-rich region; Gly, glycine-rich region; NES, nuclear export sequence; RRM, RNA-recognition motif. Full size image ARTD10 influences the activation of NF-κB reporter genes As K63-pUb is a well-known post-translational protein modification involved in NF-κB signalling, we addressed whether ARTD10 affects NF-κB function [20] . A NF-κB luciferase reporter gene stimulated by IL-1β was inhibited in a dose-dependent manner by ARTD10 in HeLa cells ( Fig. 2a ). Mutation of either the active centre in ARTD10-G888W, which is devoid of catalytic activity, or the UIMs in ARTD10-ΔUIM was not sufficient to inactivate ARTD10s effect on NF-κB activity. However, an ARTD10 double mutant (ARTD10-DM) lacking catalytic activity and the ability to bind K63-pUb, despite being expressed slightly more efficiently than wild-type ARTD10 ( Fig. 2b ), was unable to interfere with NF-κB activity. Similar results were obtained in U2OS cells after stimulation with TNFα ( Fig. 2c ). Thus, when overexpressed either the catalytic activity or the ubiquitin binding of ARTD10 is necessary to prevent the activation of NF-κB. 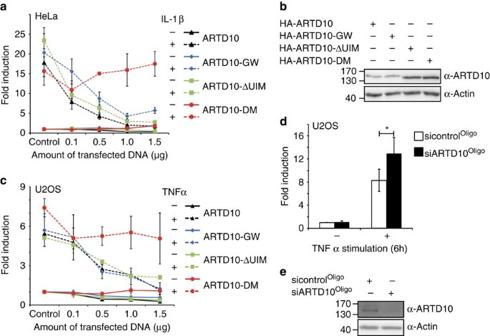Figure 2: ARTD10 interferes with NF-κB activation. (a) HeLa cells were transiently co-transfected with an NF-κB reporter plasmid and increasing amounts of plasmids encoding ARTD10, ARTD10-GW, ARTD10-ΔUIM or ARTD10-DM (combining GW and ΔUIM). The cells were serum starved overnight, stimulated with IL-1β for 6 h, lysed and luciferase activity determined. The measurements were normalized to β-Gal. Error bars represent s.d. (n=6). (b) Lysates of the experiment inawere analysed for ARTD10 expression by immunoblotting. Actin is shown for control. (c) The experiments were performed as described inabut with U2OS cells, which were stimulated with TNFα. Error bars represent s.d. (n=6). (d) U2OS cells were transiently co-transfected with an NF-κB reporter plasmid and an siRNA pool targetingARTD10mRNA. The serum-starved cells were stimulated with TNFα before the analysis of luciferase activity, which was standardized to β-Gal. Error bars represent s.d. (n=6), *P<0.05. (e) Lysates of the experiment indwere analysed for endogenous ARTD10 expression. Actin is shown for control. Figure 2: ARTD10 interferes with NF-κB activation. ( a ) HeLa cells were transiently co-transfected with an NF-κB reporter plasmid and increasing amounts of plasmids encoding ARTD10, ARTD10-GW, ARTD10-ΔUIM or ARTD10-DM (combining GW and ΔUIM). The cells were serum starved overnight, stimulated with IL-1β for 6 h, lysed and luciferase activity determined. The measurements were normalized to β-Gal. Error bars represent s.d. ( n =6). ( b ) Lysates of the experiment in a were analysed for ARTD10 expression by immunoblotting. Actin is shown for control. ( c ) The experiments were performed as described in a but with U2OS cells, which were stimulated with TNFα. Error bars represent s.d. ( n =6). ( d ) U2OS cells were transiently co-transfected with an NF-κB reporter plasmid and an siRNA pool targeting ARTD10 mRNA. The serum-starved cells were stimulated with TNFα before the analysis of luciferase activity, which was standardized to β-Gal. Error bars represent s.d. ( n =6), * P <0.05. ( e ) Lysates of the experiment in d were analysed for endogenous ARTD10 expression. Actin is shown for control. Full size image These findings were further validated by knockdown experiments in U2OS cells, which have higher endogenous ARTD10 protein levels compared with HeLa cells. The knockdown of ARTD10 with an short interfering RNA oligo pool enhanced the induction of the NF-κB reporter in response to TNFα in serum-starved cells compared with the control ( Fig. 2d ). No effect on basal activity was observed. This indicates that the endogenous ARTD10 restrains NF-κB activity upon induction. ARTD10 represses NF-κB-dependent gene and protein expression In addition to the NF-κB reporter, we determined the role of ARTD10 for the expression of chromatin-embedded target genes. Therefore, ARTD10 was transiently expressed in HeLa cells, which then were serum starved and stimulated with IL-1β. The NF-κB target genes, IκBα and IL8 , were rapidly induced while the expression of ODC1 was unaffected by IL-1β signalling ( Fig. 3a–c ). ARTD10 reduced the expression of both genes considerably, but had no effect on ODC1 messenger RNA levels. 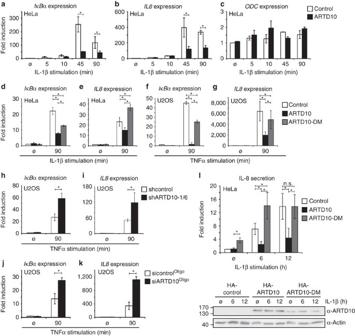Figure 3: ARTD10 inhibits IL-1β and TNFα-induced target gene expression. (a–c) HeLa cells were transiently transfected with either haemagglutinin (HA)-control or HA-ARTD10-encoding plasmids. Cells were serum starved overnight and stimulated with IL-1β. mRNA expression ofIκBα, IL8andODCwas measured by qRT-PCR and normalized toGUSexpression. Error bars represent s.d. (n=4), (d,e) HeLa cells were transiently transfected with plasmids encoding HA-ARTD10, HA-ARTD10-DM, or an empty HA plasmid for control. Cells were serum starved overnight and stimulated with IL-1β for 90 min. mRNA expression ofIκBαandIL8was analysed and normalized toGUSexpression. Error bars represent s.d. (n=4). (f,g) As described fordandebut with U2OS cells stimulated with TNFα. Error bars represent s.d. (n=4). (f,i) U2OS cells were transiently transfected with two different short hairpin RNAs targetingARTD10mRNA, andIκBαandIL8mRNA expression was analysed by qRT-PCR after 90 min of TNFα stimulation and normalized toGUS. Error bars represent s.d. (n=4). (j,k) U2OS cells were transiently transfected with an siRNA pool targetingARTD10mRNA.IκBαandIL8expression was examined as inhandI. Error bars represent s.d. (n≥4). (l) HeLa cells were transiently transfected with HA-control, ARTD10 or ARTD10-DM-encoding plasmid. Cells were serum starved overnight and stimulated with IL-1β for the indicated times. IL-8 release was measured by ELISA. The control values were set to 1, which in four independent experiments was between 3.1 and 8.5 pg ml−1of cell supernatant. For expression, control of ARTD10 cells were lysed and analysed by western blotting. Error bars represent s.d. (n=8) *P<0.05 in all experiments. Figure 3: ARTD10 inhibits IL-1β and TNFα-induced target gene expression. ( a – c ) HeLa cells were transiently transfected with either haemagglutinin (HA)-control or HA-ARTD10-encoding plasmids. Cells were serum starved overnight and stimulated with IL-1β. mRNA expression of IκBα, IL8 and ODC was measured by qRT-PCR and normalized to GUS expression. Error bars represent s.d. ( n =4), ( d , e ) HeLa cells were transiently transfected with plasmids encoding HA-ARTD10, HA-ARTD10-DM, or an empty HA plasmid for control. Cells were serum starved overnight and stimulated with IL-1β for 90 min. mRNA expression of IκBα and IL8 was analysed and normalized to GUS expression. Error bars represent s.d. ( n =4). ( f , g ) As described for d and e but with U2OS cells stimulated with TNFα. Error bars represent s.d. ( n =4). ( f , i ) U2OS cells were transiently transfected with two different short hairpin RNAs targeting ARTD10 mRNA, and IκBα and IL8 mRNA expression was analysed by qRT-PCR after 90 min of TNFα stimulation and normalized to GUS . Error bars represent s.d. ( n =4). ( j , k ) U2OS cells were transiently transfected with an siRNA pool targeting ARTD10 mRNA. IκBα and IL8 expression was examined as in h and I . Error bars represent s.d. ( n ≥4). ( l ) HeLa cells were transiently transfected with HA-control, ARTD10 or ARTD10-DM-encoding plasmid. Cells were serum starved overnight and stimulated with IL-1β for the indicated times. IL-8 release was measured by ELISA. The control values were set to 1, which in four independent experiments was between 3.1 and 8.5 pg ml −1 of cell supernatant. For expression, control of ARTD10 cells were lysed and analysed by western blotting. Error bars represent s.d. ( n =8) * P <0.05 in all experiments. Full size image Furthermore, we also measured the consequences of expressing ARTD10-DM, a poor inhibitor of the NF-κB reporter ( Fig. 2 ). Similarly, ARTD10-DM was less efficient to interfere with the expression of IκBα and showed a slight dominant negative effect on IL8 ( Fig. 3d ). Comparable experiments were performed in U2OS cells that were stimulated with TNFα. IL8 and IκBα were repressed by exogenous ARTD10 but less efficiently by ARTD10-DM ( Fig. 3f ). Finally, we measured in U2OS cells whether the presence of the endogenous ARTD10 is inhibitory for TNFα signalling. Indeed knockdown of ARTD10 using two different pSUPER constructs stimulated the expression of IL8 and IκBα ( Fig. 3h ). Enhanced expression of both genes was also observed by using an ARTD10 -specific siRNA oligo pool ( Fig. 3j ). To address whether the enhanced mRNA expression resulted in an increase in protein levels, we determined IL-8 secretion using an enzyme-linked immunosorbent assay (ELISA). HeLa cells were transiently transfected with ARTD10- or ARTD10-DM-expressing plasmids. After serum starvation the cells were stimulated with IL-1β and supernatants were analysed for IL-8. Consistent with the mRNA data, ARTD10 reduced IL-8 secretion ( Fig. 3l ). ARTD10-DM did not block IL-8 secretion but instead showed a dominant negative effect when the 6-h samples were analysed. Of note is also that we observed an increase in IL-8 secretion in serum-starved, unstimulated cells, although the mRNA level was unaffected ( Fig. 3e ). We speculate that ARTD10 might affect additional processes, including translation. This is based on findings of our substrate screen, which identified many kinases, suggesting that ARTD10 influences other signalling pathways (Feijs et al ., manuscript submitted). Together these findings suggest that ARTD10 is a negative regulator of IL-1β- and TNFα-induced signalling, most likely by affecting NF-κB. ARTD10 inhibits the nuclear translocation of p65-RelA There are different possibilities where the NF-κB signalling cascade may be regulated by ARTD10. We considered a cytoplasmic step because K63-pUb is required in the cytosol to activate NF-κB. As the signalling in the cytoplasm culminates in the translocation of the NF-κB transcription factors into the nucleus, we analysed the subcellular distribution of p65-RelA in response to IL-1β and ARTD10. Transiently transfected, serum-starved HeLa cells were stimulated with IL-1β, which induced the translocation of endogenous p65 into the nucleus within 45 min ( Fig. 4a ). ARTD10, ARTD10-G888W and ARTD10-ΔUIM reduced the translocation considerably, in accordance with their ability to inhibit NF-κB-dependent reporter gene expression. In contrast, ARTD10-DM affected only modestly the translocation of p65 ( Fig. 4a ). This is consistent with the ability of ARTD10 to reduce IL-1β-mediated degradation of IκBα in transiently transfected HeLa cells ( Fig. 4c ) and with the enhanced IκBα degradation in the presence of ARTD10-DM or upon ARTD10 knockdown ( Fig. 4c ). Together these findings indicate that indeed ARTD10 interferes with the activation of NF-κB in the cytosol. 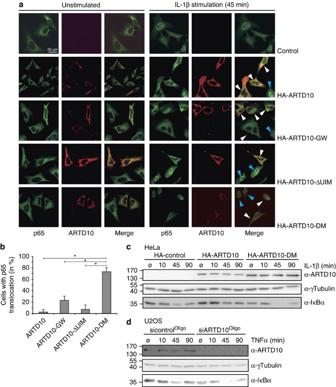Figure 4: Nuclear translocation of NF-κB p65 is blocked by ARTD10. (a) HeLa cells were transiently transfected with plasmids encoding ARTD10 and mutants. Cells were serum starved overnight. The subcellular localization of NF-κB p65 was analysed in unstimulated cells and in response to stimulation with IL-1β for 45 min. Endogenous p65 is shown in green and transiently expressed ARTD10 in red. Transfected cells in the IL-1β-treated samples are identified with white arrowheads, untransfected cells with blue arrowheads. (b) Quantification of the effects of ARTD10 and mutants on the translocation of p65. The translocation of p65 in 100–200 cells was analysed. The percentage of cells with nuclear p65 is indicated, error bars represent s.d. (four experiments with at least 50 cells analysed/condition and experiment), *P<0.05. (c) HeLa cells were transiently transfected with a control, ARTD10 or ARTD10-DM-encoding plasmid. After serum starvation overnight, the cells were stimulated with IL-1β for the indicated time points and cell lysates analysed for IκBα expression. (d) U2OS cells were transiently transfected with an siRNA pool targetingARTD10mRNA. After 48 h, the cells were serum starved overnight and stimulated with TNFα for the indicated times. Cells were lysed and IκBα protein amounts analysed by immunoblotting. Figure 4: Nuclear translocation of NF-κB p65 is blocked by ARTD10. ( a ) HeLa cells were transiently transfected with plasmids encoding ARTD10 and mutants. Cells were serum starved overnight. The subcellular localization of NF-κB p65 was analysed in unstimulated cells and in response to stimulation with IL-1β for 45 min. Endogenous p65 is shown in green and transiently expressed ARTD10 in red. Transfected cells in the IL-1β-treated samples are identified with white arrowheads, untransfected cells with blue arrowheads. ( b ) Quantification of the effects of ARTD10 and mutants on the translocation of p65. The translocation of p65 in 100–200 cells was analysed. The percentage of cells with nuclear p65 is indicated, error bars represent s.d. (four experiments with at least 50 cells analysed/condition and experiment), * P <0.05. ( c ) HeLa cells were transiently transfected with a control, ARTD10 or ARTD10-DM-encoding plasmid. After serum starvation overnight, the cells were stimulated with IL-1β for the indicated time points and cell lysates analysed for IκBα expression. ( d ) U2OS cells were transiently transfected with an siRNA pool targeting ARTD10 mRNA. After 48 h, the cells were serum starved overnight and stimulated with TNFα for the indicated times. Cells were lysed and IκBα protein amounts analysed by immunoblotting. Full size image ARTD10 prevents poly-ubiquitination of NEMO Our findings link ARTD10 to K63-pUb, a key modification to perpetuate signals generated at the IL-1β and TNFα receptors to NF-κB transcription factors. Indeed, K63-pUb of TRAF6, TAK1 and NEMO is essential for efficient signal propagation [14] , [15] , [17] . To investigate their ubiquitination, HeLa cells were co-transfected with plasmids expressing the proteins of interest, His-ubiquitin and ARTD10. These experiments were performed in the absence of proteasomal inhibitors to avoid stabilization of K48-pUb. The ubiquitinated proteins were purified using Talon beads. Ubiquitination of TRAF6 and TAK1 was enhanced in the presence of exogenous ARTD10 ( Fig. 5a ). In contrast, NEMO ubiquitination was considerably reduced in response to ARTD10 ( Fig. 5c ). Thus, TRAF6 is unlikely directly inhibited by ARTD10. As one substrate, TAK1, was ubiquitinated, it appears that NEMO poly-ubiquitination is selectively downregulated in response to ARTD10. Moreover, the enhanced poly-ubiquitination of TRAF6 and TAK1 in the presence of ARTD10 suggests that the signal is not propagated properly. The resulting reduction of NF-κB-specific gene expression is expected to inhibit the feedback capacity of the system [21] , which might prolong the stability of poly-ubiquitinated proteins upstream of the interaction point of ARTD10 with the NF-κB signalling pathway. Although the above experiments were performed in the absence of proteasomal inhibitors, we expressed a His-ubiquitin mutant, in which all lysines except K63 were replaced by arginines. Co-expression of K63only His-ubiquitin resulted in poly-ubiquitination of NEMO, which was repressed by ARTD10 ( Fig. 5d ), demonstrating that ARTD10 indeed interfered with K63-pUb. To further evaluate the role of ARTD10 in controlling the K63-pUb of NEMO, ARTD10 was knocked-down in U2OS cells and the ubiquitination of NEMO evaluated. This resulted in an enhanced NEMO K63-pUb ( Fig. 5e ), consistent with the enhanced gene expression seen above ( Fig. 3h–k ). 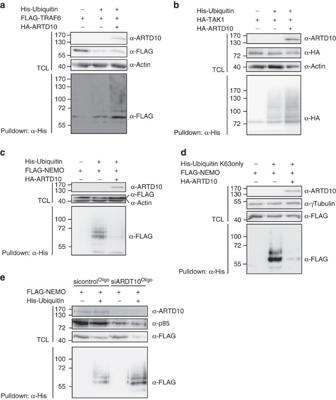Figure 5: ARTD10 prevents K63-linked poly-ubiquitination of NEMO. (a) HeLa cells were transfected with expression plasmids for FLAG-TRAF6, His-tagged ubiquitin and HA-ARTD10 as indicated. Ubiquitinated proteins were enriched on Talon beads and analysed by western blotting. TCL refers to total cell lysates in all panels. (b,c) The experiments for HA-TAK1 (b) and FLAG-NEMO (c) were performed analogous toa. (d) HeLa cells were transiently transfected with expression plasmids for FLAG-NEMO, a His-tagged ubiquitin mutant only able to form K63-linked ubiquitin polymers, and ARTD10 as indicated. The experiment was performed as described ina. (e) U2OS cells were transiently transfected with an siRNA pool targetingARTD10mRNA. The next day cells were transfected with plasmids encoding for FLAG-NEMO and His-ubiquitin as indicated. The analysis was done as ina. Figure 5: ARTD10 prevents K63-linked poly-ubiquitination of NEMO. ( a ) HeLa cells were transfected with expression plasmids for FLAG-TRAF6, His-tagged ubiquitin and HA-ARTD10 as indicated. Ubiquitinated proteins were enriched on Talon beads and analysed by western blotting. TCL refers to total cell lysates in all panels. ( b , c ) The experiments for HA-TAK1 ( b ) and FLAG-NEMO ( c ) were performed analogous to a . ( d ) HeLa cells were transiently transfected with expression plasmids for FLAG-NEMO, a His-tagged ubiquitin mutant only able to form K63-linked ubiquitin polymers, and ARTD10 as indicated. The experiment was performed as described in a . ( e ) U2OS cells were transiently transfected with an siRNA pool targeting ARTD10 mRNA. The next day cells were transfected with plasmids encoding for FLAG-NEMO and His-ubiquitin as indicated. The analysis was done as in a . Full size image ARTD10 mono-ADP-ribosylates NEMO Our results suggested a more intimate relationship between NEMO and ARTD10. Indeed NEMO and ARTD10 were coimmunoprecipitated when expressed in HEK293 cells ( Fig. 6a ). However, the interaction was weak and not detectable with endogenous proteins, with our currently available reagents. Because of the significantly diminished ubiquitination of NEMO in the presence of ARTD10 and the fact that we observed an interaction between the two proteins, we considered NEMO as an ARTD10 substrate. Indeed recombinant GST-NEMO served as substrate of ARTD10 ( Fig. 6b ). As there are currently no antibodies available currently that allow the detection of mono-ADP-ribosylated substrates, we searched for protein domains capable to bind to this modification. We have identified the macrodomains of ARTD8 as ‘reader’ modules of mono-ADP-ribosylated ARTD10 substrates [22] . Therefore, we tested whether the macrodomains of ARTD8 interacted with mono-ADP-ribosylated NEMO in vitro . Dependent on being modified by ARTD10, NEMO interacted with macrodomain 3 (Macro3) and Macro1-3 of ARTD8 ( Fig. 6c ). To define whether NEMO is also modified by ARTD10 in cells, FLAG-NEMO was transiently expressed in the presence or absence of ARTD10 or ARTD10-DM. The cell lysates were then incubated with His-Macro1-3 and the pull-downs analysed for the presence of NEMO. Only when ARTD10 was coexpressed, NEMO was capable to interact with His-Macro1-3 ( Fig. 6d ), demonstrating that NEMO is an ARTD10 substrate in cells. These findings suggested that NEMO is at least one target of ARTD10 linking mADPr to the regulation of the NF-κB signal transduction pathway. 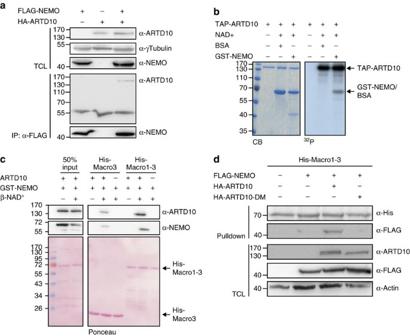Figure 6: NEMO interacts with and is substrate of ARTD10. (a) HEK293 cells were transiently transfected with plasmids encoding FLAG-NEMO and HA-ARTD10. Cells were lysed and NEMO was immunoprecipitated using FLAG beads. Western blots are shown. (b) GST-NEMO was incubated with recombinant TAP-ARTD10 protein in the presence of32P-NAD+. Radiolabelled proteins were analysed on X-ray films. The left panel depicts the Coomassie blue-stained gel (CB), on the right the autoradiography is shown (32P). (c) ADP-ribosylation assays were performed with or without TAP-ARTD10 or β-NAD+as indicated and in presence of purified GST-NEMO. The reactions were subjected to a pull-down assay with His-tagged macrodomains of ARTD8 coupled to TALON beads. Bound proteins were determined by immunoblotting (upper panels). The lower panel shows the Ponceau S staining of the blot membrane to indicate the His-tagged macrodomains. (d) HeLa cells were transiently transfected with expression plasmids for FLAG-NEMO, HA-ARTD10 or HA-ARTD10-DM as indicated. The cells were lysed and lysates used for a pull-down experiments with His-tagged mMacro1-3 coupled to TALON beads. Total cell lysates and bound proteins were analysed by western blotting. TCL refers to total cell lysates. Figure 6: NEMO interacts with and is substrate of ARTD10. ( a ) HEK293 cells were transiently transfected with plasmids encoding FLAG-NEMO and HA-ARTD10. Cells were lysed and NEMO was immunoprecipitated using FLAG beads. Western blots are shown. ( b ) GST-NEMO was incubated with recombinant TAP-ARTD10 protein in the presence of 32 P-NAD + . Radiolabelled proteins were analysed on X-ray films. The left panel depicts the Coomassie blue-stained gel (CB), on the right the autoradiography is shown ( 32 P). ( c ) ADP-ribosylation assays were performed with or without TAP-ARTD10 or β-NAD + as indicated and in presence of purified GST-NEMO. The reactions were subjected to a pull-down assay with His-tagged macrodomains of ARTD8 coupled to TALON beads. Bound proteins were determined by immunoblotting (upper panels). The lower panel shows the Ponceau S staining of the blot membrane to indicate the His-tagged macrodomains. ( d ) HeLa cells were transiently transfected with expression plasmids for FLAG-NEMO, HA-ARTD10 or HA-ARTD10-DM as indicated. The cells were lysed and lysates used for a pull-down experiments with His-tagged mMacro1-3 coupled to TALON beads. Total cell lysates and bound proteins were analysed by western blotting. TCL refers to total cell lysates. Full size image The nine postulated mono-ADP-ribosyltransferases possess a diverse combination of different domains [1] , suggesting that they will contribute to many different signalling pathways. ARTD10 is unique among these enzymes because it is the only one that has recognizable UIMs. On the basis of our observation that the UIMs of ARTD10 interact selectively with K63-pUb ( Fig. 1 ), we identified ARTD10 as a regulator of the NF-κB pathway ( Figs 2 , 3 , 4 ). Its repression is dependent on the ability of ARTD10 to interact with K63-pUb and to exert catalytic activity. ARTD10 prevents the modification of NEMO by K63-pUb, and NEMO is a target of mADPr by ARTD10 ( Figs 5 , 6 ). NEMO is a key component in the NF-κB pathway that assembles the IKK complex. This is required for upstream signalling molecules to activate IKKs and to modify IκB inhibitors. Thus, these observations provide evidence for a cross-talk between K63-pUb and mADPr by ARTD10 at a key node within the NF-κB pathway ( Fig. 7 ). 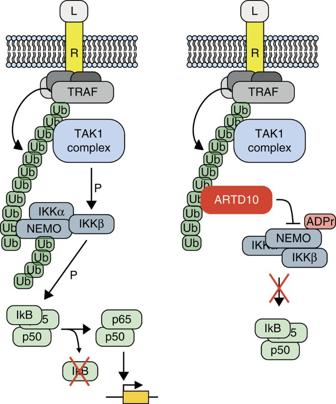Figure 7: Model of the interaction of ARTD10 with the NF-κB signal transduction pathway. ARTD10 binds to the K63-pUb and interferes with signal propagation by ADP-ribosylating NEMO and preventing NEMO K63-poly-ubiquitination. For details see text. ADPr, mono-ADP-ribosylation; IκB, inhibitor of κB; L, ligand (for example IL-1β or TNFα); NEMO (or IKKγ), NF-κB essential modulator; P, refers to a phosphorylation event; p50/p65, NF-κB transcription factor heterodimer; R, receptor; TAK1 complex, upstream activating kinase complex of IKKs; Ub, ubiquitin, the chains indicate K63-linkage. Figure 7: Model of the interaction of ARTD10 with the NF-κB signal transduction pathway. ARTD10 binds to the K63-pUb and interferes with signal propagation by ADP-ribosylating NEMO and preventing NEMO K63-poly-ubiquitination. For details see text. ADPr, mono-ADP-ribosylation; IκB, inhibitor of κB; L, ligand (for example IL-1β or TNFα); NEMO (or IKKγ), NF-κB essential modulator; P, refers to a phosphorylation event; p50/p65, NF-κB transcription factor heterodimer; R, receptor; TAK1 complex, upstream activating kinase complex of IKKs; Ub, ubiquitin, the chains indicate K63-linkage. Full size image The field of mADPr is limited at present by a lack of reagents to detect and measure this post-translational modification. There are no reliable methods to map mADPr sites. Although glutamates are the proposed sites modified by ARTD10, no formal proof has been provided. This is a general problem of cellular ADP-ribosylation, as with different mass spectrometry approaches different results were obtained for ARTD1( [23] , [24] ). Thus, although highly desirable, the modification site(s) in NEMO could not be defined for further verification and functional characterization. At present there are also no antibodies available to detect mADPr, in contrast to PAR. Recently, we have observed that the macrodomains of ARTD8 are capable to interact with mADPr ARTD10 substrates while PARylated proteins are not recognized [22] . We have now utilized this information and demonstrated that NEMO interacted with ARTD8 macrodomains upon ARTD10-dependent mADPr both in vitro and in cells. Thus, this provides evidence that NEMO is mADPr in cells, suggesting that this modification interferes with the interaction of NEMO with the upstream signalling components. This results in a lack of modification of NEMO by K63-pUb, and subsequently prevents the activation and translocation of the NF-κB transcription factor ( Fig. 7 ). The cross-talk between distinct signalling pathways is important to integrate information from different cues. Recent studies have demonstrated that ARTD5- and 6- (formerly Tankyrase1 and 2) dependent PARylation of axin results in the recruitment of the ubiquitin E3 ligase RNF146 and subsequent pUb-dependent proteasomal degradation of axin, a negative regulator of WNT signalling [9] , [10] , [25] . Similarly, 3BP2 is substrate of ARTD5 and RNF146. Mutants in 3BP2, associated with cherubism, prevent the binding of ARTD5/6 and thus reduce PARylation, leading to increased protein stability [26] , [27] . These findings define PARylation as a signal to mediate K48-linked pUb. Our findings provide an additional example for an ubiquitination–ADP-ribosylation cross-talk, although the order of events is reversed. The interaction of RNF146 with PAR appears to be primarily relevant to recruit this E3 ligase. No evidence of altered enzymatic activity has been reported. We reached similar conclusions for the interaction of ARTD10 with K63-pUb. Addition of K63-pUb did not significantly alter the catalytic activity of ARTD10 in our in vitro assays (unpublished observation). Thus, we suggest that the interaction of ARTD10 with K63-pUb serves primarily to localize ARTD10 to the K63-pUb scaffold that mediates signal propagation [19] . Once positioned at the scaffold ARTD10 may obtain access to NEMO, resulting in its mADPr and preventing further downstream signalling ( Fig. 7 ). We noticed that the overexpressed single mutants, that is, ARTD10-G888W lacking catalytic activity and ARTD10-ΔUIM missing the ability to interact with K63-pUb, were almost as efficient in inhibiting the NF-κB pathway as the wild-type protein. It is possible that ARTD10-G888W blocks signalling by binding to the K63-pUb scaffold and physically preventing other components to bind, including NEMO. Also the overexpression of ARTD10-ΔUIM may provide sufficient catalytic activity so that co-localization is less important or ARTD10 has other means to interact with NEMO, independent of K63-pUb, aspects that need to be evaluated in future experiments. Our findings suggest that ARTD10 may be part of a mechanism that modulates NF-κB signalling pathways. In this respect, it is worth noting that the expression of ARTD10 is induced in response to pathogens. For example, the treatment of peripheral blood mononuclear cells with live Borrelia burgdorferi induces the expression of ARTD10 mRNA [28] . Also the expression of ARTD10 was found upregulated in sooty mangabeys that were infected with s imian immunodeficiency virus [29] . Compatible with these findings is that ARTD10 expression is regulated by interferon-α [30] . Although these studies did not analyse whether the enhanced expression of ARTD10 affected protein level or activity, it is well possible that ARTD10 is part of feedback mechanisms that participate in terminating NF-κB signalling, thereby modulating inflammation. The NF-κB signal transduction pathway is controlled by multiple feedback mechanisms involving, for example, enzymes such as A20 and CYLD that have de-ubiquitinase activity [21] . We have analysed whether ARTD10 is directly responsive to IL-1β or TNFα. Under the conditions used here, we could not observe any increase of ARTD10 expression ( Fig. 4c ), suggesting that ARTD10 is not involved in a short-term feedback mechanism. But it may well be that ARTD10 is part of more long-term mechanisms that control NF-κB signalling. Findings in recent years have pointed to the importance of precisely controlling IL-1β or TNFα signalling by both feedback and feed-forward loops [31] . Defects in these processes have been recognized to contribute to disease, including chromic inflammation. With defining ARTD10 as a novel regulator of these pathways, the role of this enzyme and mADPr can now be addressed in both normal and pathological conditions. Cell culture and reagents U2OS and HeLa cells were kept at a humidified atmosphere at 37 °C with 5% CO 2 at all times and were cultivated in DMEM supplemented with 10% heat-inactivated fetal calf serum (FCS) and 1% penicillin/streptomycin. Transfections were performed using the calcium phosphate precipitation technique. Short hairpin RNA-mediated knockdown was achieved by co-transfection of two different pSUPER constructs targeting different regions [32] . Dharmacon siRNA pools were transfected using Lipofectamin (Invitrogen) according to the manufacturer’s instructions at a final concentration of 50 nM. The following reagents were used: Recombinant human IL-1β and TNFα (Peprotech), bio-NAD + (Trevigen), β-NAD + (Sigma), 32 P-NAD + (Perkin Elmer), recombinant human mono-ubiquitin, linear Ub 2 , K48-linked Ub 2 , K63-linked Ub 2 , K48-linked Ub (2-7) , K63-linked Ub (2–7) (Boston Biochem), glutathione-sepharose (Sigma), TALON metal affinity resin (Clontech), ANTI-FLAG M2 affinity gel (Sigma), anti-γ-tubulin (Sigma), anti-p65, anti-IκBα (Cell signaling), anti-ARTD10 (5H11) ( [3] ), anti-HA (3F10) (Roche), anti-His (H5) (Santa Cruz), anti-ubiquitin (FK-2) (Millipore), anti-GST (6G9) (provided by E. Kremmer), anti-Actin (C4) (MP Biomedicals), TAP-ARTD10 was purified as described before [3] , anti-rabbit-IgG (H+L) Alexa488-conjugated (Invitrogen), anti-rat-IgG (H+L) Alexa555-conjugated (Invitrogen). Cloning and mutagenesis Cloning of ARTD10 constructs has been described before [2] , [3] , [33] . Mutants were generated using standard mutagenesis procedures and were verified by sequencing. Cloning of pSUPER-ARTD10_1 and pSUPER-ARTD10_6 is described elsewhere [34] . Plasmids expressing FLAG-TRAF6, HA-TAK1, FLAG-NEMO, His-ubiquitin K63only and 3xNF-κB luciferase reporter constructs are described elsewhere [35] , [36] , [37] , [38] , [39] . Reporter gene assays To measure NF-κB activity, HeLa cells were seeded in 12-well plates and co-transfected the following day with the 3xNF-κB reporter gene plasmid and the indicated ARTD10-expressing plasmid. To normalize transfection efficiency, a CMV-β-galactosidase plasmid was co-transfected. Twenty-four hours after transfection, cells were starved overnight for 16 h and subsequently stimulated with IL-1β (100,000 U ml −1 ) for 6 h. Cells were lysed using extraction buffer (5 mM Tris, pH 7.8, 0.4 mM EDTA, 2% glycerol, 0.2% triton X-100, 10 mM DTT). Luciferase activities were normalized relative to β-galactosidase activities. The same procedure was performed to measure NF-κB activity in U2OS cells but by stimulating with TNFα (5 ng ml −1 ) for 6 h. Data represent three independent experiments with s.d’s. Coimmunoprecipitation For coimmunoprecipitation experiments, HEK293 cells were transiently transfected with FLAG-NEMO and HA-ARTD10. After 48 h, cells were washed with phosphate-buffered saline and collected by centrifugation. The cell pellet was resuspended in 500-μl Frackelton solution buffer (10 mM Hepes, pH 7.5, 50 mM NaCl, 30 mM NaF, 30 mM Na-pyrophosphate, 0.1 mM ZnCl 2 , protease-inhibitor cocktail). After removal of cellular debris by centrifugation for 25 min at 4 °C, a 30-μl aliquot of the lysate was used for expression control. For each immunoprecipitation 10 μl of ANTI-FLAG M2 Affinity Gel were incubated with the rest of the lysates at 4 °C under rotation for 2 h. The FLAG beads were washed three times with 1-ml Frackelton solution buffer. The precipitates and lysates were fractionated by SDS–polyacrylamide gel electrophoresis (SDS–PAGE) and subsequent western blot analysis was performed. Immunofluorescence HeLa cells were grown on coverslips (18 mm) in 12-well plates. Cells were transiently transfected with 1.5 μg of the indicated ARTD10-expressing plasmids. After 24 h, cells were starved overnight and subsequently stimulated with IL-1β (100,000U ml −1 ) for 45 min. Cells were fixed with 4% paraformaldehyde, permeabilized with 0.1% Triton X-100 and blocked in 0.2% bovine serum albumin (BSA) in phosphate-buffered saline. NF-κB p65 was stained with anti-p65 and visualized with a fluorochrome-coupled secondary antibody (Alexa-Fluor 488, anti-rabbit). HA-ARTD10 was stained with anti-HA (3F10) and visualized with a secondary antibody (Alexa-Fluor 555, anti-rat). Immunofluorescence pictures were taken by a Zeiss Axiovert 100M Confocal Laser Scanning Microscope (LSM510) equipped with an AxioCam (Zeiss) and a C-Apochromat 63x/1.2 water immersion objective. For acquisition, the software ‘LSM 510’ from Zeiss was used. For all images, the image bit depth was 12 bit and the stack size 103.01 μm × 103.01 Mm and 256 × 256 pixel. Quantitative real-time PCR HeLa or U2OS cells were transiently transfected with empty control plasmid or 1.5 μg of indicated ARTD10-expressing plasmid. Twenty-four hours after transfection, cells were starved overnight (0.1% FCS) and subsequently stimulated with IL-1β (100,000 U ml −1 ) or with TNFα (5 ng ml −1 ) for the indicated time points. Total RNA was isolated using the QIAshredder and RNeasy mini kits (QIAGEN) according to the manufacturer’s instructions. Reverse transcription was performed on 1 μg of the isolated RNA using the QuantiTect Reverse transcription kit (QIAGEN). mRNA expression levels were quantified by quantitative real-time PCR (qRT-PCR) using specific primers: IκBα forward 5′-GATCCGCCAGGTGAAGGG-3′ and reverse 5′-GCAATTTCTGGCTGGTTGG-3′; IL8 forward 5′-AGCTCTGTGTGAAGGTGCAG-3′ and reverse 5′-CCACTCTCAATCACTCTCAGC-3′; GUS forward 5′-CTCATTTGGAATTTTGCCGATT-3′ and reverse 5′-CCGAGTGAAGATCCCCTTTTTA-3′; Quantitect-Primer assay ARTD10 (QIAGEN). For ARTD10 knockdown experiments, U2OS cells were transiently transfected with pSuper-shARTD10 plasmids. Forty-eight hours after transfection, cells were starved overnight (0.1% FCS) and subsequently stimulated with TNFα (5 ng ml −1 ) for the indicated time points. In each experiment, mRNA expression of the NF-κB target genes was normalized to GUS . The statistical analyses were done using the two-sided Student’s t -test. IL-8 ELISA HeLa cells were transiently transfected with empty control plasmid or with expression plasmid encoding ARTD10 or ARTD10-DM (1.5 μg each). The cells were starved overnight (0.1% FCS) and stimulated with IL-1β (100,000 U ml −1 ) for the indicated time points. The supernatants were analysed for IL-8 by ELISA (Human IL-8 ELISA MAX Standard, BioLegend) according to the manufacturer’s instructions. Ubiquitin-binding assay GST fusion proteins were expressed in Escherichia coli BL21 cells and purified by affinity chromatography on glutathione-sepharose according to standard protocols. One microgram of purified GST-ARTD10(600–868) or GST-ARTD10(600–868)-ΔUIM was incubated with 300 ng of the indicated ubiquitin species and 30 μl of glutathione-sepharose in a reaction volume of 500 μl core buffer (50 mM NaCl, 10% glycerol, 0.1 mM EDTA, 1% NP-40, 20 mM Hepes, pH 7.5, 0.1% Triton X-100, 10 μg BSA per ml; protease-inhibitor cocktail) under rotation at 4 °C for 4 h. Beads were washed three times with 1-ml core buffer. The binding assay was separated by SDS–PAGE and analysed by western blotting. ADP-ribosylation assay ARTD10 was purified as described before [3] . ADP-ribosylation assays were carried out in 30-μl reaction buffer (50 mM Tris, pH 8.0, 0.2 mM DTT, 4 mM MgCl 2 ) with 50 μM β-NAD + and 1 μCi 32 P-NAD + or with 50 μM bio-NAD + at 30 °C for 30 min. The reactions were stopped by addition of SDS sample buffer. Reactions were fractionated by SDS–PAGE and the gels were subsequently stained with Coomassie blue. For the detection of incorporated label, the gel was exposed to X-ray films. Pull-down of mADPr-NEMO using His-Macro1-3 of ARTD8 His-Macro1-3 and His-Macro3 proteins were expressed in E. coli BL21 cells and purified by TALON Metal Affinity Resin (BD Biosciences) according to the standard protocols. For the in vitro interaction assays, 5 μg purified His-tagged macrodomains were preincubated with 25 μl equilibrated TALON beads in 350 μl IMAC lysis/wash buffer (20 mM HEPES pH 7.5, 10% glycerol, 300 mM NaCl, 0.1% NP-40, 5 mM imidazole and 14 μg ml −1 aprotinin) at 4 °C for 2 h. The binding of GST-NEMO, which was subjected to an ADP-ribosylation assay with ARTD10 in the presence or absence of NAD + , to the macrodomains was assessed by western blotting. For the interaction of cellular NEMO, HeLa cells were transiently transfected with 6 μg of FLAG-NEMO expression plasmid and 10 μg of expression plasmid for ARTD10 or ARTD10-DM. Cells were lysed in TAP-lysis buffer (50 mM Tris, pH 7.5, 150 mM NaCl, 10% glycerol, 1% NP-40). One point five micrograms of purified His-Macro1-3 were coupled to TALON beads in 50 mM NaCl, 10% glycerol, 0.1 mM EDTA, 1% NP-40, 20 mM Hepes, pH 7.5, 0.1% Triton X-100, 10 μg BSA per ml; protease-inhibitor cocktail. Protein and beads were equilibrated with TAP-lysis buffer and incubated with cell lysates at 4 °C under rotation for 1 h. Cell lysates and bound proteins were separated by SDS–PAGE and analysed by western blotting. How to cite this article: Verheugd, P. et al . Regulation of NF-κB signalling by the mono-ADP-ribosyltransferase ARTD10. Nat. Commun. 4:1683 doi: 10.1038/ncomms2672 (2013).